The actin homologue MreB organizes the bacterial cell membrane The eukaryotic cortical actin cytoskeleton creates specific lipid domains, including lipid rafts, which determine the distribution of many membrane proteins. Here we show that the bacterial actin homologue MreB displays a comparable activity. MreB forms membrane-associated filaments that coordinate bacterial cell wall synthesis. We noticed that the MreB cytoskeleton influences fluorescent staining of the cytoplasmic membrane. Detailed analyses combining an array of mutants, using specific lipid staining techniques and spectroscopic methods, revealed that MreB filaments create specific membrane regions with increased fluidity (RIFs). Interference with these fluid lipid domains (RIFs) perturbs overall lipid homeostasis and affects membrane protein localization. The influence of MreB on membrane organization and fluidity may explain why the active movement of MreB stimulates membrane protein diffusion. These novel MreB activities add additional complexity to bacterial cell membrane organization and have implications for many membrane-associated processes. The morphology of many rod-shaped bacteria is established by the coordinated incorporation of new cell wall material perpendicular to the cell axis [1] , [2] . An essential component of this machinery is the bacterial actin homologue MreB, which polymerizes into filaments at the cell periphery [3] . The peripheral association of MreB is facilitated by a conserved hydrophobic membrane-binding loop, which in some organisms is further supported by a membrane-binding N-terminal amphipathic helix [4] . Upon binding, MreB forms a complex with the conserved membrane proteins MreC and MreD, and with proteins involved in peptidoglycan synthesis such as RodA, MurG, MraY, and several penicillin-binding proteins [1] , [2] , [5] . Interference with the MreB activity renders cells mechanically less rigid [6] , and, in the absence of this, protein cells lose their rod-shaped morphology [7] , [8] . The prevailing model, in which helical MreB polymers spatially direct the synthesis of new peptidoglycan and as a result determine the general shape of the cell, has recently been revised. It turned out that MreB filaments, and the associated cell wall synthetic machinery, move around the cell in a process that is driven by peptidoglycan synthesis [9] , [10] , [11] . The MreB cytoskeleton has also been implicated in other cellular processes, including the establishment of cell polarity and chromosome segregation [12] , [13] . In a previous study, we have shown that the MreB cytoskeleton of Bacillus subtilis is sensitive to changes in the membrane potential, and incubation of cells with the proton ionophore CCCP results in a rapid delocalization of MreB [14] . The mechanism for this membrane potential sensitivity is currently unknown. During this work, we noticed that the fluorescence of the cell membrane, when stained with the lipid dye Nile Red, shows a rapid (within 1–2 min) transformation from a uniform to a clustered signal, which indicates irregularities in the lipid membrane. Interestingly, these Nile Red foci colocalize with GFP-MreB and do not emerge in bacteria that lack MreB. MreB is a homologue of eukaryotic actin, and actin forms an intricate membrane-associated network termed the cortical actin cytoskeleton [15] . The correlation between MreB and the lipid staining effects was intriguing since the cortical actin cytoskeleton is involved in the formation of lipid domains including lipid rafts and sphingolipid-enriched domains [15] , [16] . By applying different lipid staining techniques, and using a variety of mutant strains, we were able to show that the MreB cytoskeleton of B. subtilis is associated with fluid lipid domains, and, like the eukaryotic cortical actin cytoskeleton, is involved in the distribution of lipids and proteins. Furthermore, the active and directed movement of MreB appeared to stimulate the diffusion of proteins within the cell membrane. The consequences for membrane protein activity and cell wall synthesis are discussed. Altered membrane stain upon MreB delocalization Dissipation of the membrane potential with CCCP results in delocalization of the cytoskeletal protein MreB in B. subtilis [14] . We noticed that such treatment also affects fluorescent membrane staining ( Fig. 1a ). In untreated cells, Nile Red stains cell membranes without a visible preference for certain membrane areas. A slightly stronger fluorescence signal is observed for division septa, which is caused by the presence of the two adjacent cell membranes from the newly formed daughter cells. However, in the presence of CCCP, brightly fluorescent foci appear. These membrane staining effects are visible within 2 min after CCCP addition. CCCP is a proton carrier that abolishes the proton motive force (pmf)-driven synthesis of ATP, resulting in a rapid reduction of the cellular ATP pool [14] . An F 1 F o ATP synthase deletion mutant is viable and generates ATP by pmf-independent means via glycolysis and is therefore able to maintain stable ATP levels when CCCP is present for a much longer period of time [14] . Nevertheless, in an F 1 F o ATP synthase deletion strain, the addition of CCCP still results in a spotty Nile Red membrane stain, indicating that the effect is not related to changes in ATP levels ( Fig. 1b ). Addition of the potassium-ionophore valinomycin also gives rise to an irregular fluorescence membrane staining, whereas the proton-potassium antiporter nigericin has no effect ( Supplementary Fig. 1a ). Valinomycin and nigericin dissipate the membrane potential and proton gradient, respectively. Therefore, the membrane staining effects specifically occur when the membrane potential is disturbed. The presence of chloramphenicol did not prevent these effects, indicating that de novo protein synthesis is not required ( Supplementary Fig. 1b ). The fact that the fluorescent foci become visible within 1 or 2 min makes it unlikely that they are formed by local accumulation of newly synthetized membrane material. A detailed analysis of the Nile Red fluorescence spectra showed that the increased Nile Red fluorescence originates from a regular lipid bilayer environment, and is not caused by Nile Red that is bound to abnormal protein or lipid aggregates ( Supplementary Fig. 2 ). In theory, a loss of cell turgor as a result of CCCP treatment could result in the invagination of lipid membranes through plasmolysis. However, a dissipation of the membrane potential with CCCP does not cause a rapid loss of cell turgor ( Supplementary Fig. 3 ). Moreover, when the Nile Red membrane stain was compared with the fluorescent membrane signal of a GFP-labelled transmembrane protein (F 1 F o ATP synthase), the GFP signal remained unaffected by CCCP and did not correlate with the fluorescent Nile Red foci ( Fig. 1c ; Supplementary Fig. 4 ). For these reasons, we conclude that the increase in fluorescence signal is not explained by invagination of the cell membrane, or otherwise abnormal membrane shapes. 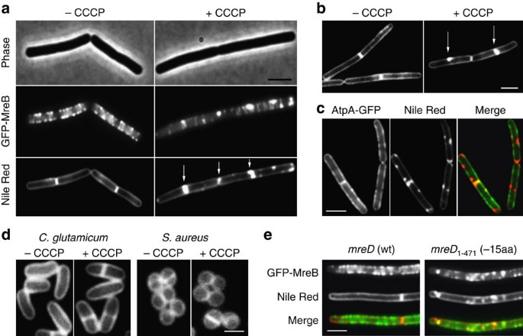Figure 1: Disruption of the MreB cytoskeleton is accompanied by an aberrant membrane stain. (a) Phase contrast images ofB. subtiliscells (upper panel) expressing GFP-MreB (middle panel), and fluorescent Nile Red membrane stains (lower panel), are depicted in the absence or presence of the proton ionophore CCCP. Some of the Nile Red foci appearing with CCCP are highlighted with arrows (seeSupplementary Fig. 5afor more examples). The CCCP-triggered local enrichment of MreB is not caused by the weak dimerization property of GFP, which was recently shown to stimulate protein clustering69(Supplementary Fig. 5b), or by artificial overproduction (Supplementary Fig. 6). Strain used:B. subtilisYK405 (gfp-mreB). (b) Incubation of F1FoATP synthase-deficient cells with CCCP also results in a rapid (within 2 min) emergence of Nile Red foci, ruling out that the appearance of Nile Red foci is due to a reduction of ATP levels (seeSupplementary Fig. 1cfor more examples). Strain used:B. subtilisHS13 (Δatp). (c) Comparison of Nile Red foci, and the localization of the integral membrane protein F1FoATP synthase fused to GFP (AtpA-GFP). The lack of overlap in fluorescence signals rules out membrane invagination, or aberrantly formed septa (see arrows) as an explanation for the strong local Nile Red fluorescence (seeSupplementary Fig. 4for more examples). The reason that in some cases the Nile red stain appears to protrude into the cytoplasm is a consequence of high membrane fluorescence originating from slightly above and below the exact focal plane. Strain used:B. subtilisBS23 (atpA-gfp). (d) CCCP does not affect Nile Red fluorescent membrane stain inStaphylococcus aureusandCorynebacterium glutamicumwhich both lack MreB (seeSupplementary Fig. 1dfor more examples). Strains used:C. glutamicumRES167 andS. aureusRN4220. (e) Colocalization of GFP-MreB (upper panel) with Nile Red (middle panel) inB. subtilisstrains encoding wild type MreD (wt), and a 15 amino acid C-terminal truncation of MreD (−15aa), which results in a mild delocalization of MreB in low Mg2+medium (seeSupplementary Fig. 1efor more examples). Strains usedB. subtilisHS35 (gfp-mreB mreDwt) and HS38 (gfp-mreB mreD1-471/−15aa). Scale bar, 2 μm. Figure 1: Disruption of the MreB cytoskeleton is accompanied by an aberrant membrane stain. ( a ) Phase contrast images of B. subtilis cells (upper panel) expressing GFP-MreB (middle panel), and fluorescent Nile Red membrane stains (lower panel), are depicted in the absence or presence of the proton ionophore CCCP. Some of the Nile Red foci appearing with CCCP are highlighted with arrows (see Supplementary Fig. 5a for more examples). The CCCP-triggered local enrichment of MreB is not caused by the weak dimerization property of GFP, which was recently shown to stimulate protein clustering [69] ( Supplementary Fig. 5b ), or by artificial overproduction ( Supplementary Fig. 6 ). Strain used: B. subtilis YK405 ( gfp-mreB ). ( b ) Incubation of F 1 F o ATP synthase-deficient cells with CCCP also results in a rapid (within 2 min) emergence of Nile Red foci, ruling out that the appearance of Nile Red foci is due to a reduction of ATP levels (see Supplementary Fig. 1c for more examples). Strain used: B. subtilis HS13 (Δ atp ). ( c ) Comparison of Nile Red foci, and the localization of the integral membrane protein F 1 F o ATP synthase fused to GFP (AtpA-GFP). The lack of overlap in fluorescence signals rules out membrane invagination, or aberrantly formed septa (see arrows) as an explanation for the strong local Nile Red fluorescence (see Supplementary Fig. 4 for more examples). The reason that in some cases the Nile red stain appears to protrude into the cytoplasm is a consequence of high membrane fluorescence originating from slightly above and below the exact focal plane. Strain used: B. subtilis BS23 ( atpA-gfp ). ( d ) CCCP does not affect Nile Red fluorescent membrane stain in Staphylococcus aureus and Corynebacterium glutamicum which both lack MreB (see Supplementary Fig. 1d for more examples). Strains used: C. glutamicum RES167 and S. aureus RN4220. ( e ) Colocalization of GFP-MreB (upper panel) with Nile Red (middle panel) in B. subtilis strains encoding wild type MreD (wt), and a 15 amino acid C-terminal truncation of MreD (−15aa), which results in a mild delocalization of MreB in low Mg 2+ medium (see Supplementary Fig. 1e for more examples). Strains used B. subtilis HS35 ( gfp-mreB mreD wt) and HS38 ( gfp-mreB mreD 1-471 /−15aa). Scale bar, 2 μm. Full size image Several experiments suggest a link between the CCCP-induced lipid staining effect and the MreB cytoskeleton. First, the Nile Red-stained membrane foci colocalize with clusters of MreB ( Fig. 1a ; Supplementary Fig. 5 ). Importantly, these clusters are not caused by artificial overproduction of a GFP-fusion protein ( Supplementary Fig. 6 ). Second, both the irregular Nile Red stain and the delocalization of MreB are triggered by valinomycin and not by nigericin [14] ( Supplementary Fig. 1a ). Third, when the effect of CCCP on Nile Red staining was tested in Staphylococcus aureus or Corynebacterium glutamicum , which do not contain MreB homologues, no change in the fluorescent membrane stain was observed ( Fig. 1d ). Finally, the localization of B. subtilis MreB depends on MreD [17] and an MreD mutant that lacks the last 15 amino acids causes an irregular MreB pattern but also an uneven Nile Red stain ( Fig. 1e ). The latter experiment indicates that the membrane staining effect occurs upon delocalization of MreB, even when the membrane potential is not affected. If the delocalization of MreB causes irregular fluorescent membrane signals, then the addition of CCCP should have no effect on the Nile Red membrane stain when MreB is absent. However, it appeared that CCCP still causes fluorescent Nile Red foci in the membrane of a B. subtilis mreB deletion mutant ( Fig. 2a ). B. subtilis encodes two other MreB homologues, Mbl and MreBH, which are known to be able to complement the activity of MreB [7] . Individual deletions of mbl or mreBH do not prevent the formation of CCCP-induced Nile Red foci either, but in the absence of all three genes (Δ mreB , Δ mbl , Δ mreBH ) the Nile Red membrane stain showed a smooth fluorescence signal in the presence of CCCP (Fig. 2a , see Supplementary Fig. 7 for the analysis of the foci frequency). Importantly, the absence of Nile Red foci in the triple mutant is not a consequence of the deformation of the cell shape by the inhibition of lateral cell wall synthesis, since inactivation of RodA, which is required for peptidoglycan synthesis in the lateral cell wall [18] , also results in round cells, yet these deformed cells still display Nile Red foci when CCCP is added ( Fig. 2b ). Taken together, these results support the suggestion that there is a correlation between MreB delocalization and the irregularities in Nile Red lipid stain. 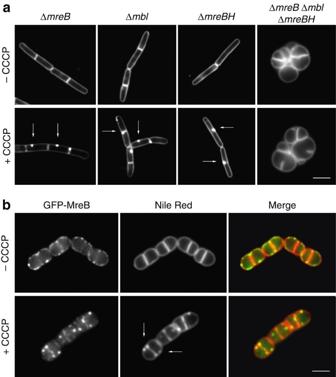Figure 2: Distorted lipid staining requires the MreB cytoskeleton. (a) CCCP-dependent fluorescent Nile Red foci occur inB. subtilisstrains deficient for single MreB homologues, but are absent in strains that lack all three MreB homologues (ΔmreB, Δmbl, ΔmreBH). Some of the Nile Red foci appearing with CCCP are highlighted with arrows. See alsoSupplementary Fig. 7for the analysis of the foci frequency. Strains used:B. subtilis3728 (ΔmreB), 4261 (Δmbl), 4262 (ΔmreBH) and 4277 (ΔmreB, Δmbl, ΔmreBH). (b) Colocalization of GFP-MreB (left panels) with Nile Red (middle panels) inB. subtiliscells depleted for RodA. The MreB cytoskeleton is disrupted with CCCP. Some of the Nile Red foci appearing with CCCP are highlighted with arrows. Strain used:B. subtilisHS36 (gfp-mreB Pspac-rodA). Scale bar, 2 μm. Figure 2: Distorted lipid staining requires the MreB cytoskeleton. ( a ) CCCP-dependent fluorescent Nile Red foci occur in B. subtilis strains deficient for single MreB homologues, but are absent in strains that lack all three MreB homologues (Δ mreB , Δ mbl , Δ mreBH ). Some of the Nile Red foci appearing with CCCP are highlighted with arrows. See also Supplementary Fig. 7 for the analysis of the foci frequency. Strains used: B. subtilis 3728 (Δ mreB ), 4261 (Δ mbl ), 4262 (Δ mreBH ) and 4277 (Δ mreB , Δ mbl , Δ mreBH ). ( b ) Colocalization of GFP-MreB (left panels) with Nile Red (middle panels) in B. subtilis cells depleted for RodA. The MreB cytoskeleton is disrupted with CCCP. Some of the Nile Red foci appearing with CCCP are highlighted with arrows. Strain used: B. subtilis HS36 ( gfp-mreB Pspac-rodA ). Scale bar, 2 μm. Full size image Involvement of specific lipids Cardiolipin (CL), phosphatidyl ethanolamine (PE) and phosphatidyl glycerol (PG) are the major phospholipid species in bacteria. Both CL and PE have been reported to form domains in B. subtilis membranes [19] , [20] . Nile Red is an uncharged fluorescent dye that partitions into lipid membranes based on its intrinsic hydrophobicity [21] , [22] . It is not known whether Nile Red prefers certain lipid head groups, but its fluorescence is sensitive to physical changes in its lipid environment [23] . To test whether an aberrant distribution of CL or PE is responsible for the irregular Nile Red stain, CL- or PE-deficient B. subtilis mutant strains were treated with CCCP. Despite the absence of CL or PE in these strains [24] , the fluorescent Nile Red foci still appear after depolarization of the membrane ( Supplementary Fig. 8a ). Another commonly used membrane dye is FM 4-64, a styryl-dye that also partitions into lipid membrane surface based on intrinsic hydrophobicity [25] . Unlike Nile Red, it does carry a positive charge [25] and a preference to bind negatively charged lipid species can be speculated. It has been shown that this dye exhibits a fluorescent stain in B. subtilis cells that under certain conditions weakly resembles a MreB-like helical pattern [26] , [27] . This was interpreted as PG-enriched helical domains since PG is negatively charged, and these structures coalesce when PG is depleted [26] , [28] . However, it turned out that this change in an FM 4-64 staining pattern is caused by depolarization of the membrane potential upon PG depletion. As in case of uncharged Nile Red, addition of CCCP readily induced FM 4-64 foci that colocalize with MreB (see Supplementary Figs 8b–e and 9 for details). Thus, we conclude that FM 4-64 is not a specific indicator for PG. The strong formation of Nile Red foci upon depletion of PG makes it unlikely that these are specific clusters of PG. Together, these results suggest that the fluorescent membrane foci are not caused by domains enriched in lipids with specific head groups. A more probable explanation for the intense fluorescent Nile Red foci is the accumulation of lipids carrying specific fatty acid species. Localization of fluid lipid domains Bacterial membranes are composed of lipids that can form different conformations such as ‘gel-phase’ or a more fluid ‘liquid-crystalline phase’. These distinct membrane configurations are predominantly determined by the fatty acid moiety of the lipids [29] , [30] . The presence of unsaturated bonds or branched chains increases the space that fatty acids occupy within a bilayer [31] . As a result, lipids containing unsaturated or branched fatty acids assemble into a more disordered ‘liquid-crystalline phase’, characterized by a less dense packing of lipids. In contrast, lipids with saturated fatty acids favour the more compact and less fluid ‘gel-phase’. The fluidity of the membrane is known to influence the fluorescent staining of many lipid dyes, including that of Nile Red [23] . To test whether this is also the case in B. subtilis cells, we measured the fluorescence intensity of Nile Red using cells that differ in their membrane fluidity. In B. subtilis the fluid lipid content is greatly altered as a response to growth temperatures. To maintain a constant membrane fluidity at different temperatures, the fluid lipid content decreases with increasing growth temperature [32] . As a consequence, when cells grown at 48 °C are cooled down to 30 °C, their cell membrane will be less fluid compared with cells that are grown at 30 °C. As shown in Fig. 3a , this results in a lower Nile Red fluorescence intensity. In contrast, if cells are grown at room temperature, and subsequently transferred to 30 °C, the membrane fluidity is increased compared with cells grown at 30 °C. Indeed, this leads to an increase in Nile Red fluorescence ( Fig. 3a ). It is therefore possible that the irregular membrane stain caused by MreB delocalization points towards local differences in membrane fluidity. 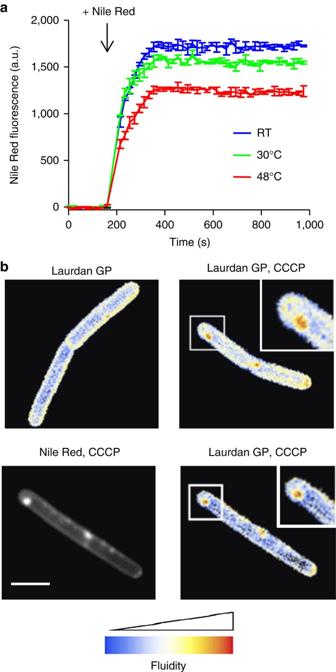Figure 3: Analysis of cell membrane fluidity. (a) Nile Red fluorescence intensity ofB. subtiliscells grown in room temperature, 30 °C or 48 °C followed by shift to 30 °C, was measured fluorometrically. To prevent rapid adaptation of membrane fluidity67, the measurements were carried out with a lipid desaturase (des)-deficient strain. The curves represent average values with s.d. of three replicate measurements. Strain used:B. subtilisHB5134 (Δdes). (b) Microscopic analysis of fluid membrane domains using Laurdan GP. The images show a colour-coded Laurdan GP intensity map in which red indicates regions of increased fluidity. Membrane fluidity is determined for untreatedB. subtiliscells (left panel) and cells treated with CCCP (right panel). See alsoSupplementary Fig. 10for the measurement of the average fluidity change. (c) Colocalization of Nile Red foci and Laurdan GP in CCCP-treatedB. subtiliscells. Strain used:B. subtilis168 (wild type). Scale bar, 2 μm. Figure 3: Analysis of cell membrane fluidity. ( a ) Nile Red fluorescence intensity of B. subtilis cells grown in room temperature, 30 °C or 48 °C followed by shift to 30 °C, was measured fluorometrically. To prevent rapid adaptation of membrane fluidity [67] , the measurements were carried out with a lipid desaturase ( des )-deficient strain. The curves represent average values with s.d. of three replicate measurements. Strain used: B. subtilis HB5134 (Δ des ). ( b ) Microscopic analysis of fluid membrane domains using Laurdan GP. The images show a colour-coded Laurdan GP intensity map in which red indicates regions of increased fluidity. Membrane fluidity is determined for untreated B. subtilis cells (left panel) and cells treated with CCCP (right panel). See also Supplementary Fig. 10 for the measurement of the average fluidity change. ( c ) Colocalization of Nile Red foci and Laurdan GP in CCCP-treated B. subtilis cells. Strain used: B. subtilis 168 (wild type). Scale bar, 2 μm. Full size image To test whether the Nile Red foci are caused by the enrichment of fluid lipids, we adapted a staining technique used to visualize fluidity differences in eukaryotic membranes. The fluidity sensitive dye Laurdan undergoes an emission wavelength shift upon changes in fluidity that can be detected microscopically [33] , [34] , [35] , [36] . As shown in Fig. 3b and Supplementary Fig. 10 , incubation with CCCP generates membrane areas with a clear and statistically significant reduction in ‘Laurdan Generalized Polarization’, which indicates an increase in local membrane fluidity. Importantly, these membrane domains colocalize with Nile Red foci ( Fig. 3c ). MreB generates membrane regions with increased fluidity These experiments suggest a direct link between the MreB cytoskeleton and membrane regions with increased fluidity (RIFs). So far, we have only observed RIFs when MreB coalesces into large clusters, and the question arises whether RIFs are present under conditions in which MreB is normally localized, rather that delocalized by CCCP or other means. Presumably, visualization of RIFs in normal uninhibited cells requires a lipid dye with a high affinity for membrane areas with increased fluidity. It has been shown that a lipid-mimicking dye DiI-C12 localizes with high specificity to fluid membrane areas as a consequence of its relative short acyl chains [37] , [38] . When B. subtilis cells were stained with this dye, a distinct punctuated fluorescent pattern became visible that overlapped significantly with the GFP-MreB signal, with a Pearson's correlation coefficient of 0.9 (Fig. 4a–c ; Supplementary Fig. 11a,b ) [37] . As a control, we tested DiI-C18, a variant with longer acyl chains. Importantly, in this case, a smooth membrane stain is observed ( Fig. 4a–c ; Supplementary Fig. 11a,b ), indicating that the fluorescent pattern of DiI-C12 is based on differences in membrane fluidity, and not a consequence of favoured interactions between the DiI head group and certain lipids or proteins. 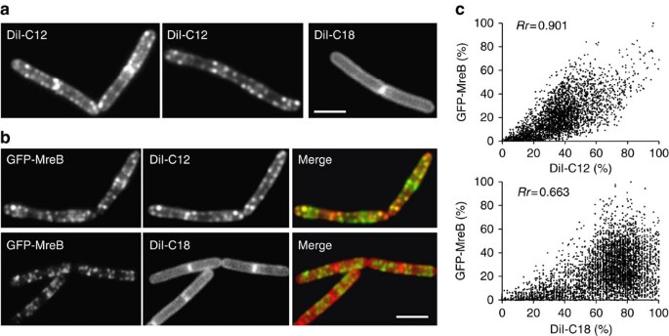Figure 4: Localization of RIFs in untreatedB. subtiliscells. (a) RIFs can be visualized in normally growing untreatedB. subtiliscells using the fluid membrane dye DiI-C12 (left panel). Staining with the long acyl-chain variant, DiI-C18, reveals a regular (smooth) membrane signal (right panel). Strain used:B. subtilis168 (wild type). (b) Colocalization of DiI-C12 and GFP-MreB (seeSupplementary Fig. 11for more examples and statistical analysis of colocalization). Strain used:B. subtilisYK405 (gfp-mreB). (c) Fluorescence intensity correlation graphs are shown for the cells in panelb. The graphs display a pixel by pixel intensity correlation between DiI and GFP-MreB fluorescence, and shows the Pearson’s correlation coefficients (Rr) (seeSupplementary Fig. 11for details). It should be mentioned that some fluorescence correlation between DiI-C18 and GFP remains since both DiI-C18 and MreB are present in the cell membrane. Strain used:B. subtilisYK405 (gfp-mreB). Scale bar, 2 μm. Figure 4: Localization of RIFs in untreated B. subtilis cells. ( a ) RIFs can be visualized in normally growing untreated B. subtilis cells using the fluid membrane dye DiI-C12 (left panel). Staining with the long acyl-chain variant, DiI-C18, reveals a regular (smooth) membrane signal (right panel). Strain used: B. subtilis 168 (wild type). ( b ) Colocalization of DiI-C12 and GFP-MreB (see Supplementary Fig. 11 for more examples and statistical analysis of colocalization). Strain used: B. subtilis YK405 ( gfp-mreB ). ( c ) Fluorescence intensity correlation graphs are shown for the cells in panel b . The graphs display a pixel by pixel intensity correlation between DiI and GFP-MreB fluorescence, and shows the Pearson’s correlation coefficients ( Rr ) (see Supplementary Fig. 11 for details). It should be mentioned that some fluorescence correlation between DiI-C18 and GFP remains since both DiI-C18 and MreB are present in the cell membrane. Strain used: B. subtilis YK405 ( gfp-mreB ). Scale bar, 2 μm. Full size image The ability to visualize RIFs with DiI-C12 without dissipation of membrane potential allowed us to test which of the MreBCD proteins are required for RIF formation. In the absence of all three MreB homologues (Δ mreB, Δ mbl , Δ mreBH ), staining with DiI-C12 produces a smooth fluorescent membrane signal, and RIFs are no longer visible ( Fig. 5a ; Supplementary Fig. 11c ). In contrast, mreC or mreD deletion strains that form comparably round cells still form RIFs ( Fig. 5a ; Supplementary Fig. 11c ), indicating that the MreB homologues rather than the integral membrane proteins MreC or MreD are essential for RIF formation. MreB can bind directly to lipid bilayers [4] , and, when GFP-MreB is expressed in a Δ mreBCD strain, a strong colocalization of GFP-MreB clusters with DiI-C12 foci is observed ( Fig. 5b ). These results show that the formation and spatial organization of RIFs is a specific property of MreB. 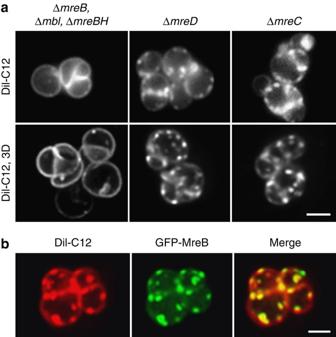Figure 5: DiI-C12-stained RIFs are MreB dependent. (a) DiI-C12 fluorescence of widefield (upper panel), and maximum intensity projection of a Z-stack (lower panel) ofB. subtilisΔmreCand ΔmreDcells, and cells that lack the three MreB homologues (ΔmreB, Δmbl, ΔmreBH). SeeSupplementary Movie 1for 3D-reconstruction,Supplementary Movie 2for corresponding raw and deconvolved images, andSupplementary Fig. 11cfor more examples. Strains used:B. subtilis3481 (ΔmreC), 4311 (ΔmreD), 4277 (ΔmreB, Δmbl, ΔmreBH, ΔrsgI). (b) Colocalization of DiI-C12 and GFP-MreB in the absence of MreBCD. The maximum intensity projections ofZ-stacks are depicted. SeeSupplementary Movie 3for 3D-reconstruction andSupplementary Movie 4for corresponding raw and deconvolved images. Strain used:B. subtilisHS35 (gfp-mreBΔmreBCD). Scale bar, 2 μm. Figure 5: DiI-C12-stained RIFs are MreB dependent. ( a ) DiI-C12 fluorescence of widefield (upper panel), and maximum intensity projection of a Z-stack (lower panel) of B. subtilis Δ mreC and Δ mreD cells, and cells that lack the three MreB homologues (Δ mreB , Δ mbl , Δ mreBH ). See Supplementary Movie 1 for 3D-reconstruction, Supplementary Movie 2 for corresponding raw and deconvolved images, and Supplementary Fig. 11c for more examples. Strains used: B. subtilis 3481 (Δ mreC ), 4311 (Δ mreD ), 4277 (Δ mreB , Δ mbl , Δ mreBH , Δ rsgI ). ( b ) Colocalization of DiI-C12 and GFP-MreB in the absence of MreBCD. The maximum intensity projections of Z -stacks are depicted. See Supplementary Movie 3 for 3D-reconstruction and Supplementary Movie 4 for corresponding raw and deconvolved images. Strain used: B. subtilis HS35 ( gfp-mreB Δ mreBCD ). Scale bar, 2 μm. Full size image Absence of MreB changes membrane properties Since MreB creates local membrane areas with increased fluidity, it might be that this activity affects the general fluidity of the cell membrane. Indeed, when the overall membrane fluidity was measured using Laurdan generalized polarization (GP), it turned out that the general membrane fluidity is significantly elevated when MreB homologues are absent ( Fig. 6a ). This increase in fluidity is comparable to the addition of 30 mM of the membrane fluidizer benzyl alcohol [39] ( Fig. 6a ). It should be added that growth in the absence of all three MreB homologues is only possible when the antisigma factor rsgI is deleted [40] , however, a Δ rsgI mutation by itself does not result in altered membrane fluidity ( Fig. 6a ). Δ mreC or Δ mreD strains show identical changes in cell shape and inhibition of lateral cell wall synthesis as the triple mreB mbl mreBH deletion mutant but still contain RIF clusters. Importantly, the overall membrane fluidity of these strains is comparable to wild-type cells. 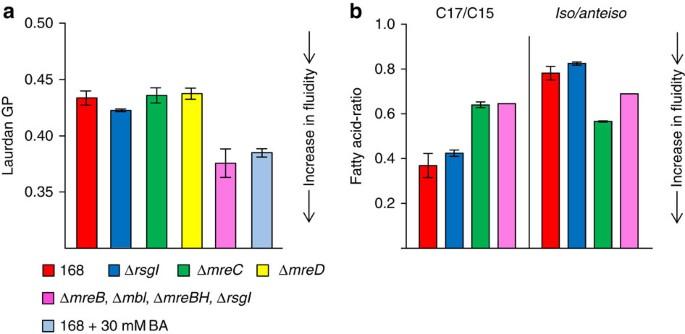Figure 6: Membrane fluidity increases in the absence of MreB. (a) Overall membrane fluidity of several cytoskeletal mutant strains was measured as Laurdan GP of logarithmically growingB. subtiliscells. As a positive control, an increase in fluidity (= decrease in Laurdan GP) was established by adding the membrane fluidizer benzyl alcohol (BA; 30 mM) to wild type cells. The diagram depicts the average values and s.d. of three independent measurements. (b) Ratios between chain lengths of the major fatty acids (C17 and C15) and ratios between theisoandanteisoforms of fatty acids are depicted for the different strains (seeSupplementary Table 1for the detailed composition). High C17/C15 or highiso/anteisoratios indicate a reduced fluidity. The diagram depicts the average values and s.d. of two independent analyses. Strains used:B. subtilis168 (wild type), 4264 (ΔrsgI), 3481 (ΔmreC), 4277 (ΔmreB, Δmbl, ΔmreBH, ΔrsgI). Figure 6: Membrane fluidity increases in the absence of MreB. ( a ) Overall membrane fluidity of several cytoskeletal mutant strains was measured as Laurdan GP of logarithmically growing B. subtilis cells. As a positive control, an increase in fluidity (= decrease in Laurdan GP) was established by adding the membrane fluidizer benzyl alcohol (BA; 30 mM) to wild type cells. The diagram depicts the average values and s.d. of three independent measurements. ( b ) Ratios between chain lengths of the major fatty acids (C17 and C15) and ratios between the iso and anteiso forms of fatty acids are depicted for the different strains (see Supplementary Table 1 for the detailed composition). High C17/C15 or high iso/anteiso ratios indicate a reduced fluidity. The diagram depicts the average values and s.d. of two independent analyses. Strains used: B. subtilis 168 (wild type), 4264 (Δ rsgI ), 3481 (Δ mreC ), 4277 (Δ mreB , Δ mbl , Δ mreBH , Δ rsgI ). Full size image The Laurdan experiments suggest that RIFs formed by MreB affect the overall fluidity. However, it is possible that the absence of MreB influences the actual lipid composition. To investigate this, the fatty acid compositions of the different strains were analysed using gas chromatography ( Fig. 6b ; Supplementary Table 1 ). Both the Δ mreC mutant and mreB triple mutant (Δ mreB/mbl/mreBH ) increase their overall fatty acid chain length (less C15 and more C17 species), which normally lowers the membrane fluidity ( Fig. 6b ; Supplementary Table 1 ). The Δ mreC , and to a lesser extent the mreB triple mutant, also increases the fraction of ‘ anteiso ’ fatty acids compared with ‘ iso ’ fatty acid species. Anteiso fatty acid species carry a methyl group attached to the third last carbon of the chain and are significantly more fluid than iso species, which carry a methyl group attached to the second last carbon [41] . In case of Δ mreC , this increase in anteiso fatty acids seems to compensate for the effect of increased fatty acid chain length since the overall membrane fluidity of this Δ mreC mutant is the same as for wild type ( Fig. 6a ). Importantly, this increase in anteiso fatty acids is lower in the mreB triple mutant compared with the Δ mreC mutant ( Fig. 6b ; Supplementary Table 1 ), and yet the overall fluidity of the MreB triple mutant is significantly higher ( Fig. 6a ). The strong increase of membrane fluidity of the mreB triple mutant can therefore not be explained by an altered fatty acid composition. This suggests that the MreB protein complex concentrates fluid lipids into RIFs, which results in lower overall membrane fluidity. These experiments provide further evidence for the specific role of MreB homologues in maintaining a proper lipid homeostasis in the cell membrane. MreB is important for membrane protein distribution The cortical actin cytoskeleton is involved in segregation of the eukaryotic cell membrane into domains that differ in fluidity, including the formation of lipid rafts [15] , [16] , [42] , [43] , [44] , [45] . This activity of actin influences the localization and diffusion of many membrane proteins [46] , [47] , [48] , [49] , [50] . Since MreB is an actin homologue and creates distinct membrane domains, the question arises whether the MreB cytoskeleton also influences the distribution of membrane proteins. To test this, the MreB cytoskeleton was disrupted with CCCP, and the localization of several integral membrane proteins was analysed. Indeed, incubation with CCCP induces clustering of several membrane proteins including Fructose permease (FruA), P16.7, YhaP and YqfD and RNase Y ( Fig. 7a ). Other proteins, such as succinate dehydrogenase (SdhA) and F 1 F o ATP synthase (AtpA), showed no apparent difference in localization pattern ( Fig. 7a ). The proteins FruA, YhaP, P16.7 and YqfD show a clear clustering with Nile Red foci in CCCP-treated cells ( Supplementary Fig. 12 ). To test whether this clustering depends on MreB, and is not caused by CCCP itself, we analysed the localization of these proteins in the mreB triple mutant strain. Indeed, in this strain background, the localization of these proteins was unaffected by CCCP ( Fig. 7b ). Thus, the MreB-induced fluid lipid domains can influence the distribution of membrane proteins. It should be added that the localization pattern of RNase Y is still influenced by dissipation of membrane potential in MreB triple mutant ( Fig. 7b ), suggesting that in this case the effect is MreB independent. 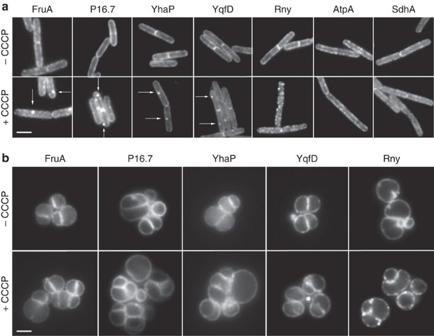Figure 7: Aberrant localization of different membrane proteins. (a) The localization of several membrane proteins (FruA, P16.7, YhaP, YqfD and Rny) is changed after the MreB cytoskeleton was disturbed by addition of CCCP. Some of the foci appearing with CCCP are highlighted with arrows. The localization of other proteins (AtpA and SdhA) remains unaffected. SeeSupplementary Fig. 12for more examples, and colocalization with Nile Red. Strains used:B. subtilisFruA-GFP, 110WA (p16.7-gfp),yhaP-gfp, yqfD-gfp, 3569 (rny-gfp), BS23 (atpA-gfp), BS112 (sdhA-gfp). (b) The CCCP-induced clustering of membrane proteins FruA, P16.7, YhaP and YqfD is absent in strains deficient for MreB homologues. Strains usedB. subtilisHS43 (rny-gfp, ΔmreB*), HS44 (fruA-gfp, ΔmreB*), HS45 (P16.7-gfp, ΔmreB*), HS46 (yhaP-gfp, ΔmreB*), HS47 (yqfD-gfp, ΔmreB*).mreB*designates (ΔmreB, Δmbl, ΔmreBH, ΔrsgI). Scale bar, 2 μm. Figure 7: Aberrant localization of different membrane proteins. ( a ) The localization of several membrane proteins (FruA, P16.7, YhaP, YqfD and Rny) is changed after the MreB cytoskeleton was disturbed by addition of CCCP. Some of the foci appearing with CCCP are highlighted with arrows. The localization of other proteins (AtpA and SdhA) remains unaffected. See Supplementary Fig. 12 for more examples, and colocalization with Nile Red. Strains used: B. subtilis FruA-GFP, 110WA ( p16.7-gfp ), yhaP-gfp, yqfD-gfp , 3569 ( rny-gfp ), BS23 ( atpA-gfp ), BS112 ( sdhA-gfp ). ( b ) The CCCP-induced clustering of membrane proteins FruA, P16.7, YhaP and YqfD is absent in strains deficient for MreB homologues. Strains used B. subtilis HS43 ( rny-gfp , Δ mreB* ), HS44 ( fruA-gfp , Δ mreB* ), HS45 ( P16.7-gfp , Δ mreB* ), HS46 ( yhaP-gfp , Δ mreB* ), HS47 ( yqfD-gfp , Δ mreB* ). mreB* designates (Δ mreB , Δ mbl , Δ mreBH , Δ rsgI ). Scale bar, 2 μm. Full size image MreB stimulates membrane protein diffusion The MreB complexes of B. subtilis move rapidly along the cell membrane, driven by the cell wall synthesis machinery. This movement can be slowed down by inhibiting peptidoglycan synthesis with vancomycin [9] , [10] . Since MreB affects the localization of lipids and membrane proteins, it is possible that the active movement of MreB also influences the diffusion dynamics of membrane proteins. To test this, the diffusion of several membrane proteins was followed using high-speed total internal reflection (TIRF) microscopy. As shown in the kymographs of Fig. 8a , the diffusion dynamics of FruA and F 1 F o ATP synthase changed significantly when the movement of MreB was stopped with vancomycin. The same behaviour was observed for two other tested transmembrane proteins ( Supplementary Fig. 13a , see also Supplementary Fig. 13b for quantitation based on fluorescence intensity fluctuation). 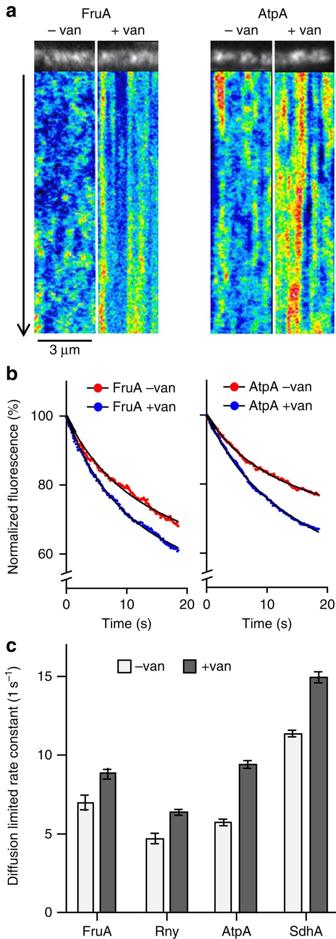Figure 8: MreB movement influences membrane protein diffusion. (a) Kymographs visualizing the diffusion of fructose permease (FruA) and F1FoATP synthase (AtpA) in the absence and presence of vancomycin (van), which blocks MreB movement. Time lapse series with 20 s length and 100 ms time resolution was acquired using TIRF microscopy. SeeSupplementary Movie 5for corresponding raw image series. (b) In TIRF microscopy, only proteins within the vicinity of the evanescent light (<200 nm distance from the coverslip surface) are subject to fluorophore (GFP) bleaching. The graphs depict the averaged, normalized and background-subtracted fluorescent signals of fructose permease (FruA) and F1FoATP synthase (AtpA) in the presence (− van) and absence (+ van) of MreB movement. A significant increase in bleaching is observed when movement of MreB is inhibited with vancomycin, which indicates a reduced diffusion of proteins in and out of the range of the evanescent light. The curve fits were performed using a two-phase exponential decay model composed of a rapid bleaching of GFP within the range of the evanescent wave, and slower (diffusion limited) bleaching of the whole cell fluorescence (seeSupplementary Fig. 14for details). (c) Rate constants and s.e. of slow (diffusion limited) bleaching kinetics for Fructose permease (FruA), RNaseY (Rny), F1FoATP synthase (AtpA) and Succinate dehydrogenase (SdhA) in the absence and presence of vancomycin. Increased rate constant indicates a reduced exchange of protein between the TIRF-illuminated area and rest of the cell surface. The number of analysed cells, goodness-of-fit and s.e. are provided inSupplementary Fig. 14. Strains used:B. subtilisBS23 (atpA-gfp), BS112 (sdhA-gfp), FruA-GFP and 3569 (rny-gfp). Figure 8: MreB movement influences membrane protein diffusion. ( a ) Kymographs visualizing the diffusion of fructose permease (FruA) and F 1 F o ATP synthase (AtpA) in the absence and presence of vancomycin (van), which blocks MreB movement. Time lapse series with 20 s length and 100 ms time resolution was acquired using TIRF microscopy. See Supplementary Movie 5 for corresponding raw image series. ( b ) In TIRF microscopy, only proteins within the vicinity of the evanescent light (<200 nm distance from the coverslip surface) are subject to fluorophore (GFP) bleaching. The graphs depict the averaged, normalized and background-subtracted fluorescent signals of fructose permease (FruA) and F 1 F o ATP synthase (AtpA) in the presence (− van) and absence (+ van) of MreB movement. A significant increase in bleaching is observed when movement of MreB is inhibited with vancomycin, which indicates a reduced diffusion of proteins in and out of the range of the evanescent light. The curve fits were performed using a two-phase exponential decay model composed of a rapid bleaching of GFP within the range of the evanescent wave, and slower (diffusion limited) bleaching of the whole cell fluorescence (see Supplementary Fig. 14 for details). ( c ) Rate constants and s.e. of slow (diffusion limited) bleaching kinetics for Fructose permease (FruA), RNaseY (Rny), F 1 F o ATP synthase (AtpA) and Succinate dehydrogenase (SdhA) in the absence and presence of vancomycin. Increased rate constant indicates a reduced exchange of protein between the TIRF-illuminated area and rest of the cell surface. The number of analysed cells, goodness-of-fit and s.e. are provided in Supplementary Fig. 14 . Strains used: B. subtilis BS23 ( atpA-gfp ), BS112 ( sdhA-gfp ), FruA-GFP and 3569 ( rny-gfp ). Full size image In TIRF microscopy, a major determinant is the diffusion of GFP in and out of the range of the evanescent light. The reduction in membrane protein diffusion should thus increase photobleaching. Indeed, for all tested proteins, a significant increase in diffusion-limited GFP bleaching was observed in the presence of vancomycin ( Fig. 8b,c ; Supplementary Fig. 14 ). Thus, the active movement of the MreB cytoskeleton stimulates diffusion of membrane proteins. Despite their small size, the cell membrane of bacteria exhibits a remarkably complex organization. There are lipid species that accumulate at cell division sites and cell poles, and most membrane proteins are not uniformly distributed over the bacterial cell membrane [30] , [51] , [52] . In addition, it has been reported that B. subtilis can form low fluidity ‘lipid rafts’ [53] , [54] , [55] . The capacity of the MreB cytoskeleton to induce fluid lipid domains (RIFs) that determine the distribution of membrane proteins adds a new dimension to this complexity. The mechanism through which MreB organizes fluid lipids remains hypothetical. Peripheral membrane proteins have a capacity to induce lipid domains [56] , [57] . This activity is related to the binding of lipid bilayers by means of an intercalating amphipathic helix, but these domains are absent in MreB homologues from Gram-positive bacteria [4] . However, it has also been postulated that peripheral membrane proteins can directly induce fluid lipid domains by reducing the ordering effect of electrostatic attraction and repulsion between charged lipid head groups [58] . Although this mechanism is in good agreement with the electrostatic membrane-binding mode of MreB [4] , we cannot rule out the involvement of other MreB-interacting proteins in the formation of RIFs. Because of the various cellular functions of the cytoplasmic membrane, an organization into membrane areas that differ in their physical properties has a clear advantage. The optimal fluid state of the membrane is a compromise between different factors. On the one hand, high membrane fluidity promotes protein activity by reducing viscosity, and thus stimulating catalytic activity and diffusion of integral membrane proteins [59] . A higher membrane elasticity of fluid membranes also allows the lipid bilayer to optimally embed membrane proteins [60] , [61] . On the other hand, high membrane fluidity has the disadvantage that it increases proton permeability [32] , [62] , resulting in a less efficient energy and ion homeostasis. The MreB-dependent formation of fluid lipid domains (RIFs) could therefore enable the cell to maintain an optimal condition for membrane protein activity in limited areas of increased fluidity without compromising the proton permeability of the whole membrane. In a recent study, it was shown that the random motion of chromosomes in bacterial and yeast cells is faster than that can be explained by simple Brownian motion. This increased molecular diffusion rate is caused by ATP-dependent processes such as RNA synthesis [63] . This bears some similarity with our observation that the diffusion of membrane proteins is also stimulated by an active process, in this case peptidoglycan synthesis, and the subsequent movement of RIFs. It is tempting to speculate that the continuous mixing of the cell membrane by active RIF movement promotes diffusion of proteins in a viscous membrane environment, thereby stimulating protein–protein and protein–substrate interactions. Inactivation of MreB prevents lateral cell wall synthesis resulting in deformed round cells. This effect can be explained by the inability to recruit the necessary proteins to the proper site of synthesis. However, the fluid membrane environment created by MreB might also be required for optimal cell wall synthesis since Lipid II, the membrane-anchored precursor for peptidoglycan synthesis, has a strong preference for fluid membranes [64] . Possibly, RIFs are enriched with this essential precursor. In fact, the delocalization of MreB with CCCP does coincide with a loss of lateral Lipid II localization, based on staining with fluorescently-labelled vancomycin, whereas staining of the cell division septum remains unaffected ( Supplementary Fig. 15 ). With its ability to organize lipids and proteins in the bacterial cell membrane, MreB bears a functional resemblance to the eukaryotic cortical actin cytoskeleton [15] , [42] , [44] , [45] . There are, however, differences. The actin cytoskeleton forms a relatively static meshwork at the membrane periphery [65] , yet the bacterial counterpart is more fragmented [9] , [10] , [11] . In eukaryotic cells, the membrane-anchored actin creates fences that restrict diffusion of proteins [65] , whereas the active movement of the MreB cytoskeleton stimulates diffusion. Interestingly, it was recently shown that short and highly dynamic actin polymers, which influence clustering of membrane proteins, also exist in eukaryotic cells [48] . Thus, despite some differences, the ability of MreB and actin to induce and organize membrane domains appears comparable, and may explain why actin and MreB are evolutionarily linked. Strains and growth conditions The growth conditions and construction of strains are described in the Supplementary Materials and Methods. The used strains and conditions for gene induction are listed in Supplementary Table 2 . General fluorescence microscopy For fluorescence microscopy, cells were grown to exponential growth phase at 30 °C if not stated otherwise. The cells were immobilized on microscope slides covered with a thin film of 1.2% agarose in water. For the dissipation of membrane potential with CCCP, the mounting medium was supplemented with 0.5% dimethylsulphoxide (DMSO) or 100 μM CCCP dissolved in DMSO (0.5% final concentration of DMSO). Imaging was carried out within 2 min after addition of ionophores. Membranes were visualized with Nile Red or FM 4-64 (0.5 μg ml −1 ). Standard fluorescence microscopy was carried out using Zeiss Axiovert 200 M (Zeiss Plan-Neofluar × 100/1.30 Oil Ph3 objective), Nikon Eclipse Ti (Nikon Plan Fluor × 100/1.30 Oil Ph3 DLL objective), and Applied Precision DeltaVision RT (Zeiss Plan-Neofluar 100x/1.30 Oil Ph3) microscopes. The images were acquired with Metamorph 6 (Molecular Devices), softWoRx Suite (Applied Precision), and further analysed using ImageJ v.1.38 (National Institutes of Health). Deconvolution was carried from optical sections using Huygens Essentials v.3.3 (Scientific Volume Imaging). Laurdan GP microscopy For the microscopic analysis of membrane fluidity, B. subtilis cells grown in LB medium were incubated for 5 min with 100 μM Laurdan, washed and then resuspended in fresh prewarmed LB. No inhibitory effect on growth was detected with 100 μM Laurdan. Laurdan was exited at 360±20 nm, and fluorescence emission was captured at 528±19 nm (exposure time: 500 ms) followed by a second image at 457±25 nm (exposure time: 500 ms). Image analysis and generation of a colour-coded GP map were performed with Wolfram Mathematica 7 (Wolfram Research). In brief, the background fluorescence was subtracted, and GP values were calculated for each pixel, based on intensities values of the separate images, as GP=( I 457 − I 528 )/( I 457 + I 528 ), whereby I 457 represents the emission intensity at 457±25 nm and I 528 emission intensity at 528±19 nm. To remove signals not associated with cells, pixel pairs were regarded as insignificant when one of the channel intensities was below a threshold of 10% of the maximal values found in the membrane. Insignificant pixel pairs were assigned a GP of zero. Finally, GP pixel values were represented as a linear colour-coded GP map, whereby blue represents high GP values (low fluidity) and red represents low GP values (high fluidity). Insignificant pixels (GP=0) are shown in black. The full Wolfram Mathematica-script can be obtained from the authors upon request. The ability of the microscope-based assay to detect changes in membrane fluidity was verified by measuring changes in membrane fluidity upon cold shock or incubation with 30 mM benzyl alcohol [66] ( Supplementary Fig. 16a ). For the measurement of mean GP values, the membrane fluorescence signal intensities at both emission channels were extracted as maximum values from a fluorescence intensity line scan perpendicular to the membrane plane. The values were measured for 70 individual cells, background subtracted, and the Laurdan GP values were calculated as described above. To prevent fast adaptation of membrane fluidity, a B. subtilis strain deficient for lipid desaturase (Δ des ) was used in this case [67] . Des itself has no influence on the appearance of RIFs upon incubation with CCCP ( Supplementary Fig. 16b ). Laurdan GP spectroscopy For the measurement of membrane fluidity in batch cultures, cells were grown in LB supplemented with 0.1% glucose to an OD 600 ~0.5, followed by 5 min incubation with 10 μM Laurdan. Subsequently, cells were washed three times with prewarmed buffer containing 50 mM Na 2 HPO 4 /NaH 2 PO 4 pH 7.4, 0.1% glucose and 150 mM NaCl with and without the membrane fluidizer benzyl alcohol (30 mM). In case of the different Mre-mutant strains, the media and buffers were supplemented with 20 mM MgCl 2 . The Laurdan fluorescence intensities were measured at 435±5 nm and 490±5 nm upon excitation at 350±10 nm, using a Tecan Infinite 200 M fluorometer. The Laurdan GP was calculated using the formula GP=( I 435 − I 490 )/( I 435 + I 490 ). In both microscopic and spectroscopic measurements, the Laurdan GP assay was able to reliably detect general changes in membrane fluidity, although, due to different excitation and emission wavelengths used, the absolute values obtained with microscopy slightly differed from the normal batch fluidity measurements ( Supplementary Fig. 16a ). The fluorescence emission spectrum of Laurdan was recorded using 10 μM Laurdan embedded in liposomes upon excitation with 350 nm light using a Tecan Infinite 200 M fluorometer. The liposomes were formed from E. coli polar lipids using detergent dialysis method. In brief, the lipid extract was solved in chloroform followed by evaporation under dry argon stream. The lipids were resolubilized in 25 mM Tris/HCl pH 7.4 and 1.5% octylglucoside (25 mg ml −1 lipids), followed by dialysis against 25 mM Tris/HCl pH 7.4. At last, the formed liposomes were diluted to 1:5 in H 2 0 and sized by extrusion through a 0.1-μm membrane. DiI-C12 staining of fluid lipid domains For staining of B. subtilis cells with DiI-C12, an overnight culture was diluted 1:100 in medium supplemented with 5 μg ml −1 DiI-C12 and 1% DMSO followed by growth for 2.5 h at 30 °C. Because of the high fluorescence of unbound dye, the stained cells were washed three times in prewarmed medium supplemented with 1% DMSO, followed by microscopy. The staining of B. subtilis with DiI-C18, which is insoluble in water, was carried out by suspending small amounts of solid DiI-C18 crystals in culture medium followed by 2.5 h incubation at 30 °C, based on a method described in Kim et al . [68] For microscopy, the crystals were removed by a brief low speed centrifugation. No growth inhibitory effect of the Dil-dyes was observed ( Supplementary Fig. 17 ). For colocalization studies, the concentration of DiI-C12 was reduced to 2.5 μg ml −1 . The reason for this was the extensive overlap of the excitation spectra between DiI-C12 and GFP, which results in weak GFP fluorescence. The emission spectra of GFP and Dil-C12 are well separated, and no significant bleach-through of the emitted fluorescence was detected for DiI-C12 in the GFP channel, and vice versa . TIRF time lapse microscopy The analysis of membrane protein diffusion was carried out using a Nikon Eclipse Ti equipped with, Nikon CFI APO TIRF × 100/1.49 Oil objective, TIRF illumination module, Andor Xion X 3 EMCCD-camera and 488 nm solid state laser. The cells were imaged for 20 s with 100 ms time resolution in a continuous illumination mode. The image analysis including the generation of kymographs was carried out using ImageJ v.1.38 (National Institutes of Health) and Multiple Kymograph plugin (J. Rietdorf and A. Seitz). TIR-CP analysis For the analysis of GFP-bleaching kinetics upon TIRF illumination, the average fluorescence intensity of cells was measured using an automated detection of cell area based on above background fluorescence intensity (ImageJ v.1.38, National Institutes of Health). In brief, the cell detection was performed using the first image frame and subsequently used to measure the average fluorescence intensity for each image of the time series. The background fluorescence signals were extracted from the same images as the average intensity of the remaining image area not associated with cells. The background subtracted and normalized intensity values were used to fit the GFP photobleach kinetics as mono- or biexponential decays using GraphPad Prism 5 (GraphPad Software). The fixation of GFP, applied to inhibit diffusion was performed by incubation of the cell samples with paraformaldehyde for 5 min at RT, followed by saturation of formaldehyde crosslinking by the addition of 100 mM Glycine. Spectral imaging fluorescence microscopy The analysis of the emission wavelength spectrum for Nile Red-stained B. subtilis cells was carried out with Nikon A1R point scanning confocal microscope using Nikon Plan Apo VC × 60 NA 1.4 oil objective and 561 nm excitation laser. The emission spectrum was recorded with a 4.8-nm window size for the total range of 570–749 nm. Image analysis was carried out with NIS-Elements 4.0 (Nikon). Membrane fluidity-dependent Nile Red fluorescence intensity Nile Red exhibits low fluorescence in a polar environment such as LB, but emits strongly when incorporated into hydrophobic cell membranes. This property was used to measure the intensity of Nile Red membrane fluorescence in B. subtilis cells grown in LB at different growth temperatures. For this, growing cultures were diluted to an optical density of OD 600 =0.5. Subsequently, the temperature of the cultures was rapidly adjusted to 30 °C, and the fluorescence increase was measured after addition of 0.5 μg ml −1 Nile Red. The measurements were carried out at 30 °C using a BMG Fluostar Optima fluorometer, and 584 nm excitation, and 620 nm emission filters. Background fluorescence was subtracted using signals measured from Nile Red in LB. To prevent rapid adaptation of membrane fluidity [67] , the measurements were carried out with a lipid desaturase-deficient strain ( B. subtilis Δ des ). Analysis of fatty acid composition The fatty acid composition of B. subtilis wild-type cells and the cytoskeletal mutants was determined from cells grown at 30 °C in LB supplemented with 20 mM MgCl 2 that were collected when the cultures reached an OD 600 of approximately 0.5. Fatty acids were analysed as fatty acid methyl esters using gas chromatography. All analyses were carried out in duplicates by the Identification Service of the DSMZ, Braunschweig, Germany. How to cite this article: Strahl, H. et al . The actin homologue MreB organizes the bacterial cell membrane. Nat. Commun. 5:3442 doi: 10.1038/ncomms4442 (2014).